Downsizing a human inflammatory protein to a small molecule with equal potency and functionality A significant challenge in chemistry is to rationally reproduce the functional potency of a protein in a small molecule, which is cheaper to manufacture, non-immunogenic, and also both stable and bioavailable. Synthetic peptides corresponding to small bioactive protein surfaces do not form stable structures in water and do not exhibit the functional potencies of proteins. Here we describe a novel approach to growing small molecules with protein-like potencies from a functionally important amino acid of a protein. A 77-residue human inflammatory protein (complement C3a) important in innate immunity is rationally transformed to equipotent small molecules, using peptide surrogates that incorporate a turn-inducing heterocycle with correctly positioned hydrogen-bond-accepting atoms. Small molecule agonists (molecular weight <500 Da) examined for receptor affinity and cellular responses have the same high potencies, functional profile and specificity of action as C3a protein, but greater plasma stability and bioavailability. Protein–protein interactions underlie most biological processes defining life, aging, disease and death. However, the use of proteins in science, industry and medicine is still significantly restricted by their high cost of manufacture, chemical instability, immunogenicity and poor bioavailability. The need to overcome these deficiencies has driven many chemical efforts, but it has been extremely challenging to reproduce the exquisitely potent and specific actions of proteins [1] , [2] , [3] , [4] , [5] , [6] . The biological functions of some proteins are localized in very short polypeptide segments stabilized in specific structures (two to four helical turns, isolated β-turns, strands/sheets, and their combinations) by their protein environments [7] , [8] . Yet, even in these simpler cases, short synthetic peptides corresponding to bioactive protein components do not display functional potencies comparable to proteins and are not thermodynamically stable structures in water, where they instead adopt random interconverting structures [9] . An important example of a protein to functionally mimic is the human complement protein C3a. This is a 9 kDa helix bundle that plays key roles in innate immune responses to infection and tissue injury by interacting with a 100 kDa cell surface protein, a G protein-coupled receptor (GPCR) called C3aR [10] , [11] , [12] . C3a is a powerful pro-inflammatory agent that recruits immune cells to sites of infection (chemotaxis) and induces immune cells to secrete bactericidal agents (via degranulation) as well as inflammatory cytokines [13] , [14] . Overexpression of C3a/C3aR or sustained activation of its receptor can lead to inflammatory diseases, including allergies [10] , asthma [15] , arthritis [16] , sepsis [17] , lupus [18] , diabetes [19] , psoriasis [20] , nephropathy [21] , ischaemia-reperfusion injury [22] , obesity, and metabolic and cardiovascular dysfunction [23] . C3a also reportedly has antimicrobial [24] and antifungal [25] activities. Despite these potent activities, C3a is rapidly degraded in vivo to C3a-desArg [26] , which has a different pharmacology from C3a and does not bind to C3aR [27] , nor do commercially available antibodies discriminate between C3a and C3a-desArg [22] . Synthetic agonists that act through C3aR, but do not degrade as C3a does, can be expected to have immunostimulating and degranulating activities, whereas stable antagonists may be valuable new anti-inflammatory therapeutics. However, despite decades of effort by academia and the pharmaceutical industry, no small organic molecules have yet been reported as potent and selective C3aR agonists or antagonists [28] , [29] , [30] , [31] , [32] . The crystal structure of C3a [33] , [34] , [35] reveals that its 77 amino acids adopt a well-defined helix bundle ( Fig. 1a ), with less structure in carboxy-terminal residues known to be critical for receptor activation [36] . Mutagenesis of C3a and its receptor support a two-site binding model [37] . The helical bundle residues 1–69 of C3a have high affinity for (but do not activate) the receptor, through multiple positive-charged lysine and arginine residues of C3a making complementary interactions with negative-charged Asp residues in the unusually large extracellular loop 2 (ECL2) at one site of the C3aR [38] , [39] . On the other hand, the C-terminal pentapeptide segment LGLAR of C3a has very low affinity for a second site on C3aR, leading to activation. Arg77 at the C- terminus of C3a is critical for agonist activity; on removal, the resulting C3a-desArg does not bind to C3aR [27] . Moreover, mutagenesis of Arg161, Arg340 and Asp417 in the receptor has shown these residues to be crucial for C3a binding and activation [40] . The essential Arg77 residue is the only charged residue near the C terminus of C3a and is thought to interact with the above three charged residues of C3aR. 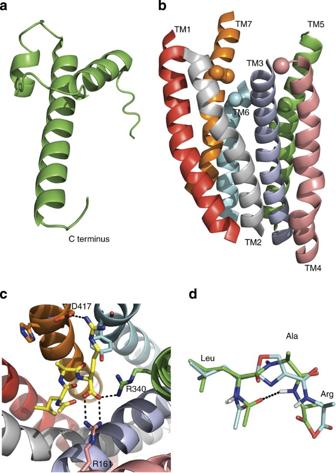Figure 1: Modelling C3aR interactions with Leu–Ala–Arg. (a) Structure of human C3a (pdb 4I6O). (b) Side view of seven transmembrane (7TM) region of C3aR homology model derived from the crystal structure of human CXCR4 (bound to a cyclic peptide antagonist)41. Cα of D417, R161, R340, H418 and Y393 rendered as solid spheres. (c) Ac–Leu–Ala–Arg (3, yellow) placed in the 7TM region of human C3aR, showing putative interactions with receptor residues D417 (TM7), R161 (TM4) and R340 (TM5) identified from mutagenesis38,39,40to be important for binding to Arg77 of C3a. (d) A low-energy conformation of Ac–(Leu–Ox)–Arg (6, cyan carbons; Ox, oxazole) aligned well with Ac–Leu–Ala–Arg (3, green carbons) modelled in a type IIβ turn conformation (φi+1−60°,ψi+1120°,φi+280°,ψi+20°), showing the typical (i,i+3) H-bond Ac–CO…HN–Arg (Arg side chains omitted for clarity). Figure 1: Modelling C3aR interactions with Leu–Ala–Arg. ( a ) Structure of human C3a (pdb 4I6O). ( b ) Side view of seven transmembrane (7TM) region of C3aR homology model derived from the crystal structure of human CXCR4 (bound to a cyclic peptide antagonist) [41] . Cα of D417, R161, R340, H418 and Y393 rendered as solid spheres. ( c ) Ac–Leu–Ala–Arg ( 3 , yellow) placed in the 7TM region of human C3aR, showing putative interactions with receptor residues D417 (TM7), R161 (TM4) and R340 (TM5) identified from mutagenesis [38] , [39] , [40] to be important for binding to Arg77 of C3a. ( d ) A low-energy conformation of Ac–(Leu–Ox)–Arg ( 6 , cyan carbons; Ox, oxazole) aligned well with Ac–Leu–Ala–Arg ( 3 , green carbons) modelled in a type IIβ turn conformation ( φ i+1 −60°, ψ i+1 120°, φ i+2 80°, ψ i+2 0°), showing the typical (i,i+3) H-bond Ac–CO…HN–Arg (Arg side chains omitted for clarity). Full size image Here we exemplify the approach of growing a functionally important amino acid of a protein, namely the arginine from the C-terminus of C3a, into small molecules that can execute the potent functions of the C3a protein, but are only a fraction of the size, cheaper to synthesize, and more chemically and biologically stable. We describe small molecules built from an amino acid template, incorporating a specific heterocycle to make important hydrogen bonds (H-bonds) with the C3a receptor and to control the shape of the molecule and orientation of its hydrophobic substituents. The small molecules have similar affinity for C3aR on human macrophages and comparable agonist potencies and functional profiles to C3a, as measured by intracellular calcium release and inflammatory gene expression in human macrophages and degranulation of human mast cells. Importantly, the small molecule agonists are stable in serum, unlike C3a that rapidly degrades with loss of the C-terminal arginine that is critical for binding of C3a to its receptor C3aR. If generally applicable, this template approach could potentially be useful in creating small molecule surrogates of other proteins for applications in biology and medicine. C3aR homology model and ligand evolution We therefore created a three-dimensional homology structural model for C3aR ( Fig. 1b ) and positioned only an arginine amino acid into C3aR in the vicinity of those three receptor residues ( Fig. 1c ). A homology model of the human C3a receptor was generated, using the Prime module in the Schrödinger molecular modelling suite, based on aligning its sequence with that of the crystal structure of human chemokine receptor CXCR4 (bound to a cyclic peptide antagonist) [41] (pdb code 3OE0). Models were created to focus on the seven transmembrane (7TM) helix domain, without the ECL2, which in C3aR consists of 170 amino acids and is inherently flexible and difficult to model ( Fig. 1b ). An arginine molecule was specifically placed in this model, near receptor residues Arg161, Arg340 and Asp417, to simulate Arg77 of the C3a ligand. The negatively charged carboxylate terminus of Arg77 in C3a interacts with cationic side chains of both Arg161 and Arg340, whereas the protonated guanidinium side chain of Arg77 interacts with the carboxylate side chain of Asp417 ( Fig. 1c ). These three contact points are consistent with C3aR/C3a mutagenesis data, indicating complementarity between Arg77 in C3a and the above three residues of C3aR [38] , [39] , [40] . On the basis of this location for Arg77, we identified space that could be occupied by attached amino acids Ala76 and Leu75 of C3a, thereby indicating where a small tripeptide ligand LAR might bind in C3aR. This was the basis for our strategy to rationally design and grow novel small molecule ligands from an arginine point template corresponding to Arg77 of C3a, notwithstanding the large uncertainties of ligand docking in a three-dimensional model of a GPCR. Structure–activity relationships Tripeptides Leu–Ala–Arg ( 2 ), Ac–Leu–Ala–Arg ( 3 ) and Boc–Leu–Ala–Arg ( 4 ) did not show any detectable binding to C3aR or agonist activity at or below 1 mM, the highest concentration tested, on human monocyte-derived macrophages (HMDMs) ( Table 1 ). Next, we sought to establish whether there were residues present in the 7TM-binding cavity and/or the ECLs that could potentially form additional H-bonding interactions with the backbone of Leu or Ala from the tripeptide Leu–Ala–Arg. Three receptor residues were conspicuous as prospective H-bond donors in the proximity of the Ala attached to Arg, namely Tyr393 from TM6 and His418 from TM7 ( Fig. 1c ), and possibly Tyr174 from ECL2, although the latter position is very uncertain owing to ECL2 flexibility. Although GPCR models are notoriously flexible and thus of uncertain accuracy, we decided to test whether H-bond acceptors strategically placed at the Ala position might increase affinity for C3aR, thereby confirming the idea that an H-bond donor might be nearby its binding site in C3aR. Ala in Leu–Ala–Arg was therefore replaced with oxazole (Ox), which positions a known H-bond-accepting nitrogen atom of Ox within (Leu–Ox)–Arg for potential interaction with a putative H-bond donor Tyr393, His418 or Tyr174. This ligand change from Leu–Ala–Arg ( 2 ) to (Leu–Ox)–Arg ( 5 ) resulted in a >1,000-fold increase in affinity for C3aR and some measurable, albeit weak, agonist activity ( Table 1 ). Importantly, structure–activity optimization does not rely on knowing the identity of the interacting H-bond donor in C3aR. 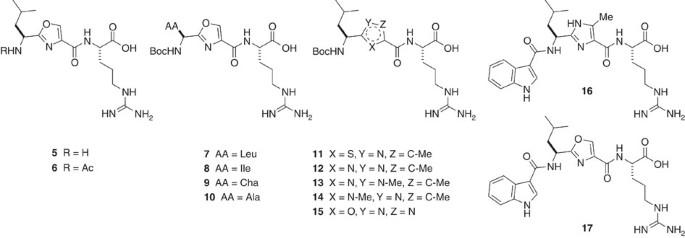Figure 2: Synthesised C3aR ligands. Chemical structures of compounds5–17, synthesized as detailed in the Methods (16,17) andSupplementary Methods(5–15). Figure 2 details the chemical structure of ligand 5 and further modified ligands 6 – 17 to be discussed below. Table 1 Binding affinity and agonist potency of ligands for C3aR on human macrophages. Full size table Figure 2: Synthesised C3aR ligands. Chemical structures of compounds 5 – 17 , synthesized as detailed in the Methods ( 16 , 17 ) and Supplementary Methods ( 5 – 15 ). Full size image The magnitude of the increase in affinity cannot be accounted for solely by one H-bond to the Ox, and is in part also attributed to the known turn-inducing constraint imposed by this heterocycle, conferring some structure in water to an otherwise unstructured tripeptide unit. Most peptide-activated GPCRs bind to a β/γ-turn conformation of endogenous agonists [42] , and incorporation of a turn mimetic often pre-organizes agonists in a receptor-bound turn conformation. An alignment using ROCS (rapid overlay of chemical structures, version 3.1.2, OpenEye Scientific Software) of low-energy conformers generated with Omega (version 2.4.3, OpenEye Scientific Software) of Ac–Leu–Ala–Arg ( 3 ) with Ac–(Leu–Ox)–Arg ( 6 ) indicated that a β-turn conformation of the former was mimicked by the latter ( Fig. 1d ). The plane of the Ox ring is perpendicular to the plane of the Leu amide carbonyl, favourably aligning for making a H-bond interaction ( Fig. 1d ). In support of formation of this additional H-bond, attaching a carbonyl group to the amino terminus of 5 (for example, Ac in Ac–(Leu–Ox)–Arg, 6 ; Boc in Boc–(Leu–Ox)–Arg, 7 ) caused ~20- and ~50-fold increases in ligand affinity for C3aR and ~10 3 -fold greater agonist activity than for 5 ( Table 1 ). In combination, these data support both the heterocycle nitrogen and the N-terminal carbonyl oxygen being important H-bond acceptors that contribute to the spectacular increase in receptor binding and agonist function. Modifying side chains and heterocycles Further modifications of the leucine side chain to isoleucine ( 8 ) caused a 3-fold loss of affinity, to the larger side chain of cyclohexylalanine ( 9 ) reduced binding affinity 8-fold and agonist potency 3-fold, whereas reducing the size of the side chain to alanine ( 10 ) reduced affinity and agonist activity by over 1,000-fold. Thus, the leucine side chain is important and essential for binding to C3aR and contributes a factor of at least 10 3 to agonist binding and function. On the basis of the promising results for Ox in compound 7 , other five-membered aromatic heterocycles were incorporated to identify the contribution of the heterocycle H-bond acceptor to agonist potency. The theoretical H-bond interaction energy between a water molecule and each heterocycle was determined using models minimized by ab initio methods at the MP2/6 311++g(3d,3p) level of theory using Gaussian 09 (ref. 43 ). Strong interactions were predicted for the trigonal nitrogen atoms of imidazole and Ox rings, whereas much weaker H-bonds are likely for the oxygen of oxadiazole and sulphur or π system of thiazole. N -methylation in the inactive compound 14 precluded H-bond formation, so the H-bond interaction energy was set at zero ( Fig. 3a ). For this small series of heterocycles incorporated into Boc–Leu–Ala–Arg to produce compounds 7 and 11 – 15 , there was a linear correlation between H-bond interaction energy (over a 35 kJ mol −1 range), calculated for the respective H-bond acceptor interacting with water, and the binding affinity (over 4 log units) of the ligand for C3aR ( Fig. 3b,c ). Positioning of the H-bond-accepting atom was an important determinant of agonist potency, the X position being more important than Y or Z positions ( Table 1 ), highlighted by the N -methyl imidazole substituents in 13 versus 14 . 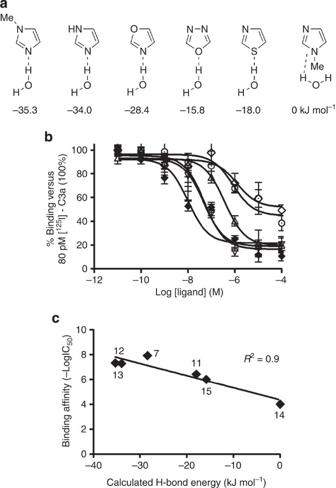Figure 3: Effect of heterocycles on ligand binding to C3aR. (a) Calculated (MP2/6-311++g(3d,3p)) (ref.43) H-bond interaction energy (kJ mol−1) predicted between water and a heteroatom of heterocycles. (b) C3aR-binding affinty of compounds7(black diamonds, oxazole),11(triangles, thiazole),12(inverted triangles, imidazole),13(cross, NMe(Y)-imidazole),14(circle, NMe(X)-imidazole),15(white diamonds, oxadiazole) measured by competition with [125I]-C3a (80 pM) in HMDMs. Error bars are means±s.e.m. (c) Linear correlation between C3aR-binding affinity (−LogIC50) and calculated H-bond interaction energy (kJ mol−1) predicted for water binding to different heterocyclic compounds7and11–15. Figure 3: Effect of heterocycles on ligand binding to C3aR. ( a ) Calculated (MP2/6-311++g(3d,3p)) (ref. 43 ) H-bond interaction energy (kJ mol −1 ) predicted between water and a heteroatom of heterocycles. ( b ) C3aR-binding affinty of compounds 7 (black diamonds, oxazole), 11 (triangles, thiazole), 12 (inverted triangles, imidazole), 13 (cross, NMe(Y)-imidazole), 14 (circle, NMe(X)-imidazole), 15 (white diamonds, oxadiazole) measured by competition with [ 125 I]-C3a (80 pM) in HMDMs. Error bars are means±s.e.m. ( c ) Linear correlation between C3aR-binding affinity (−LogIC 50 ) and calculated H-bond interaction energy (kJ mol −1 ) predicted for water binding to different heterocyclic compounds 7 and 11–15 . Full size image Having identified imidazole and Ox as optimal heterocycle modifications, the N-terminal Boc group was next replaced to seek greater agonist potency. The indole-3-carboxamide derivatives 16 and 17 showed approximately threefold greater binding affinity and almost tenfold greater agonist activity than 12 and 7 , respectively. These observed enhancements may be due to the indole ring making an additional π -stacking interaction with His418 and occupying a larger region of hydrophobic space in the C3a receptor. Concentration–response curves are compared ( Fig. 4a ) for C3a versus the most potent small molecule agonist above, compound 17 (also named TR16), in the intracellular Ca 2+ release assay using HMDMs. It is apparent that 17 shows a full agonist response comparable to C3a, but that 17 is almost an order of magnitude more active (EC 50 (half maximal effective concentration) 7 nM versus 40 nM). Moreover, this agonist activity for both C3a and 17 was dose-dependently inhibited to the same degree by a known, albeit weakly potent antagonist of C3aR (SB290157, IC 50 (half maximal inhibitory concentration) 1 μM versus C3a at 1 μM) [28] , [29] , consistent with the effect being mediated in both cases by C3aR ( Fig. 4b ). The high agonist potencies of 17 and C3a are, in spite of their quite different affinities for C3aR ( Fig. 4c ), the much greater affinity of C3a being due to its additional large helical domain that binds to an extracellular region of the receptor. The presence of this high-affinity receptor-anchoring domain in C3a provides a high effective molarity for the receptor-activating C-terminus of C3a, which is otherwise a weakly binding and very feeble agonist (compound 1 , Table 1 ). Altering concentrations of both 17 and SB290157 (ref. 29 ) revealed competition between the compounds, evidenced by a horizontal shift to the right in agonist plots ( Fig. 4d ), with a Schild plot slope ~1 ( Fig. 4e ) consistent with both compounds binding to the same or overlapping site on C3aR. An important advantage of compound 17 over C3a is that 17 remains intact after exposure to plasma, whereas the arginine is cleaved from C3a within minutes in plasma ( Fig. 4f ) by carboxypeptidases [26] . The product of this cleavage is C3a-desArg, which has quite a different pharmacology and a different receptor [44] ; thus, C3a is actually of little value as a tool to probe C3aR-mediated functions induced in vivo by constitutive C3a. The plasma stability of small molecule agonists such as 17 is likely to be of enormous benefit for in vivo studies, provided that they display other comparable functional responses to C3a, and can therefore be used as small molecule surrogates for C3a (see ahead). 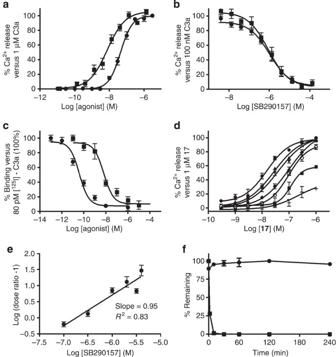Figure 4: Affinity and Ca2+mobilization for C3a versus 17. (a) iCa2+mobilization induced in HMDMs by compound17(squares) versus C3a (circles) at various concentrations, relative to 100% fluorescence for 1 μM C3a (n≥3). Agonist17is >5-fold more potent than C3a. (b) SB290157 inhibits intracellular Ca2+release induced in HMDMs by either C3a (circles, 100 nM) or compound17(squares, 100 nM), with comparable inhibitory potency (IC501.0 μM,n≥3). (c) C3aR-binding affinities of compound17(squares) versus C3a (circles) measured by displacement of125I-C3a (80 pM) (n>3), the higher affinity of the latter owing to the additional helical domain of C3a. (d) Concentration–response for agonist17±antagonist SB290157 at various concentrations (zero, closed circles; 0.1 μM, triangles; 0.3 μM, inverted triangles; 1.0 μM, diamonds; 2.0 μM, squares; 3 μM, open circles; 4 μM cross;n=3). (e) Schild plot (slope=0.95) of data fromFig. 4d, indicating competitive inhibition of17by SB290157. (f) Unlike C3a (not shown),17(circles) was intact in rat plasma after 4 h (at 37 °C, pH 7.4, initial concentration 1 μM), whereas linear peptide4(squares) was rapidly degraded and undetectable after 10 min, as measured by liquid chromatography mass spectroscopy (LCMS) (n=3). Error bars are means±s.e.m. Figure 4: Affinity and Ca 2+ mobilization for C3a versus 17. ( a ) iCa 2+ mobilization induced in HMDMs by compound 17 (squares) versus C3a (circles) at various concentrations, relative to 100% fluorescence for 1 μM C3a ( n ≥3). Agonist 17 is >5-fold more potent than C3a. ( b ) SB290157 inhibits intracellular Ca 2+ release induced in HMDMs by either C3a (circles, 100 nM) or compound 17 (squares, 100 nM), with comparable inhibitory potency (IC 50 1.0 μM, n ≥3). ( c ) C3aR-binding affinities of compound 17 (squares) versus C3a (circles) measured by displacement of 125 I-C3a (80 pM) ( n >3), the higher affinity of the latter owing to the additional helical domain of C3a. ( d ) Concentration–response for agonist 17 ±antagonist SB290157 at various concentrations (zero, closed circles; 0.1 μM, triangles; 0.3 μM, inverted triangles; 1.0 μM, diamonds; 2.0 μM, squares; 3 μM, open circles; 4 μM cross; n =3). ( e ) Schild plot (slope=0.95) of data from Fig. 4d , indicating competitive inhibition of 17 by SB290157. ( f ) Unlike C3a (not shown), 17 (circles) was intact in rat plasma after 4 h (at 37 °C, pH 7.4, initial concentration 1 μM), whereas linear peptide 4 (squares) was rapidly degraded and undetectable after 10 min, as measured by liquid chromatography mass spectroscopy (LCMS) ( n =3). Error bars are means±s.e.m. Full size image Profiling additional agonist functions Compound 17 was thus also compared with recombinant human C3a for other functional agonist responses using different assays and different cells. 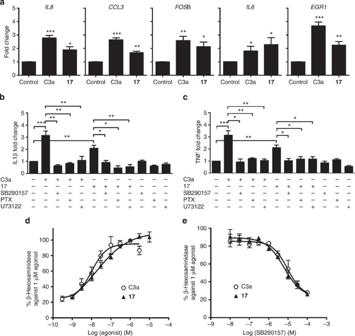Figure 5: Inflammatory gene expression and degranulation induced by C3a versus 17. (a) C3a or17(0.3 μM, 30 min) induce expression of inflammatory genes in HMDMs, monitored by quantitative reverse-transcriptase PCR. Relative gene expression data are duplicates normalized to housekeeping gene18S. Fold changes were calculated against untreated control. Error bars represent mean±s.e.m. of at least three independent experiments. *P<0.05; **P<0.01; ***P<0.005. (b,c) Expression in HMDMs of inflammatory genesIL1βandTNFinduced by C3a or17(0.3 μM, 30 min) alone or after preincubating cells with C3aR antagonist (10 μM SB290157, 30 min), Gαi inhibitor (200 ng ml−1pertussis toxin (PTX), overnight) or PLCβ inhibitor (10 μM U73122, 30 min). (d,e) β-Hexosaminidase release mediated by C3a (pEC508.0±0.3) and17(pEC507.8±0.6) in the absence or presence of SB290157 in LAD2 human mast cells. Cells were pre-sensitized with IgE (100 ng ml−1, overnight) before adding C3a (1 μM at 1.5 log dilutions) or17(10 μM at 1.5 dilutions) for 30 min. In the antagonist assay, cells sensitized overnight with IgE were incubated with SB290157 (100 μM at 1.5 log dilutions, 30 min) before adding C3a or17(1 μM) for 30 min. Release of β-hexosaminidase in cell supernatant and lysate was detected by adding p-nitrophenylN-acetyl-β-D-glucosamide (PNAG) and reading absorbance at 405 nm. % β-Hexosaminidase release was calculated against response for 1 μM agonist. Error bars represent mean±s.e.m. of (n=4) independent experiments. Figure 5a–c shows that C3a and 17 induce comparable profiles of expression of the inflammatory genes IL8 , CCL3 , FOSB , IL6 and EGR1 in HMDMs. Moreover, IL1β and TNF gene expression induced by either C3a or 17 was blocked by the known [29] , but very weakly potent C3aR antagonist SB290157, by pertussis toxin that decouples C3aR from Gi, and by the PLCβ inhibitor U73122 that blocks C3aR-mediated Ca 2+ release ( Fig. 5b,c ). These effects are consistent with the actions of 17 being mediated through C3aR and point to comparable potencies with C3a in the responses being measured. Finally, in different human immune cells, both C3a and 17 at nM to μM concentrations induced degranulation of human mast cells to the same extent, as measured by comparable release of hexosaminidase ( Fig. 5d ). Further, this agonist response was inhibited to the same extent for C3a and 17 by SB290157 ( [29] Fig. 5e ). These data give very strong support for compound 17 being a viable, equipotent, functional surrogate for the human C3a protein. We expect that this compound class can be further developed into valuable drug-like agonists and antagonists for treating C3aR-mediated diseases. Figure 5: Inflammatory gene expression and degranulation induced by C3a versus 17. ( a ) C3a or 17 (0.3 μM, 30 min) induce expression of inflammatory genes in HMDMs, monitored by quantitative reverse-transcriptase PCR. Relative gene expression data are duplicates normalized to housekeeping gene 18S . Fold changes were calculated against untreated control. Error bars represent mean±s.e.m. of at least three independent experiments. * P <0.05; ** P <0.01; *** P <0.005. ( b , c ) Expression in HMDMs of inflammatory genes IL1β and TNF induced by C3a or 17 (0.3 μM, 30 min) alone or after preincubating cells with C3aR antagonist (10 μM SB290157, 30 min), Gαi inhibitor (200 ng ml −1 pertussis toxin (PTX), overnight) or PLCβ inhibitor (10 μM U73122, 30 min). ( d , e ) β-Hexosaminidase release mediated by C3a (pEC 50 8.0±0.3) and 17 (pEC 50 7.8±0.6) in the absence or presence of SB290157 in LAD2 human mast cells. Cells were pre-sensitized with IgE (100 ng ml −1 , overnight) before adding C3a (1 μM at 1.5 log dilutions) or 17 (10 μM at 1.5 dilutions) for 30 min. In the antagonist assay, cells sensitized overnight with IgE were incubated with SB290157 (100 μM at 1.5 log dilutions, 30 min) before adding C3a or 17 (1 μM) for 30 min. Release of β-hexosaminidase in cell supernatant and lysate was detected by adding p-nitrophenyl N -acetyl-β- D -glucosamide (PNAG) and reading absorbance at 405 nm. % β-Hexosaminidase release was calculated against response for 1 μM agonist. Error bars represent mean±s.e.m. of ( n =4) independent experiments. Full size image A method has been described for downsizing a protein to an equipotent functional small molecule, a method that does not require a crystal structure for the protein but does rely on some knowledge of the activating region of the protein. The C3a protein chosen here for mimicry has its functional activity localized at its C-terminus, but requires the remainder of the protein for high affinity binding to the receptor to elicit agonist activity and high potency. In this study, the high affinity binding domain of C3a has been removed, but compensated for by making rational changes to small molecule mimics of the C-terminal tripeptide segment of C3a, namely Leu–Ala–Arg. These changes impart H-bond-accepting properties, introduce a turn-inducing heterocycle and enhance space-filling properties of the small molecule analogues. The results convincingly demonstrate that a number of compounds ( 7 , 8 , 13 , 16 and 17 ) have equipotent agonist activity to the protein C3a, as measured by induction of intracellular Ca 2+ release in human macrophages ( Table 1 ). The most potent compound ( 17 ) was examined in more detail in other cellular assays, with mimicry of potent C3a function also extending to C3aR-mediated expression of all seven selected inflammatory genes in human macrophages and to C3aR-mediated degranulation of human mast cells. These immunostimulating properties for 17 are the same as for human C3a, validating successful functional mimicry of a protein by a small molecule across a range of inflammatory and cellular readouts. Through structure–activity relationships, it has been shown that six factors contribute to the spectacular agonist potencies of these compounds, which are approximately six orders of magnitude more potent than the Leu–Ala–Arg tripeptide component of C3a but are not much different in size. (1) These compounds possess an important arginine, just like the critical C-terminal arginine of human C3a, which imparts some binding affinity for C3aR. (2) All compounds possess an Ox or imidazole heterocycle, which also provides (3) a strong H-bond-accepting nitrogen atom, as well as (4) subtly altering the position of the Leu/Ile side chain in the dipeptide surrogate (Leu/Ile–heterocycle) versus Leu/Ile–Ala. These compounds further share (5) the presence of an N-terminal carbonyl group that can make an additional H-bond interaction with C3aR and (6) a Boc/Indole capping group that can fill additional space in the receptor. The relative contributions made by each of these components to ligand affinity and agonist potency were ascertained via structure–activity relationship studies ( Table 1 ). Collectively, these features have led to the rational development of small molecules (molecular weight <500 Da) with high affinity and specificity for the human C3a receptor and comparable agonist potencies to C3a. The most potent compound was profiled more extensively in multiple additional assays where it was found to have the same C3aR-mediated functional profile, selectivity, activities and potencies as human C3a protein. Compound 17 was shown to be a potent and C3aR-selective agonist surrogate for C3a ( Supplementary Fig. S5 ), with the advantage of being plasma stable unlike C3a, which rapidly loses its C-terminal arginine along with its affinity for and function through the receptor for C3a. Moreover, all the small molecules described herein can be made at a fraction of the thousands of dollars per milligram cost commercially charged for human C3a. This approach to potent small molecule protein mimics may be transferable to the development of highly potent small molecule mimics of other proteins, including other GPCR-activating proteins. It is based on a very general premise, that one may only need to know that an amino acid of a protein (arginine here) is important for binding at a particular site on a receptor protein, in this case through known effects on the donor protein of site-directed mutagenesis of the receptor protein. This single amino acid can then be grown through a novel method of appending a H-bond-making entity, heterocycles with graded H-bond acceptor versus H-bond donor properties being chosen here to illustrate the idea. In principle, this H-bond making appendage could be placed anywhere, on one side or the other side, or both sides of the arginine (or other point template) or further away. On finding measurable affinity, the putative H-bond interaction can be rationally optimized by increasing the H-bonding power, then by modifying the next position adjacent to the heterocycle–arginine motif to rationally improve binding and optimize function. Although only exemplified here for one protein, this is a potentially general approach. It remains to be determined whether its utility is also general for developing small molecules with the functional potencies of other proteins. General methods All reagents were purchased from Sigma-Aldrich or Chem-Impex International Inc. Solid- and solution-phase chemistry approaches were used to synthesize all final compounds. The purity of each compound investigated was confirmed by 1 H NMR spectroscopy, HPLC and high-resolution mass spectra (HRMS). All compounds assayed were ≥95% pure. The syntheses and characterization of compounds 2 – 15 are reported in Supplementary Methods and reaction schemes and spectroscopic data are provided in Supplementary Figs S2–S20 . The production and characterization of the two most potent compounds, 16 and 17 , are described below. All final compounds were purified by reversed-phase HPLC. Preparative-scale reversed-phase HPLC (rpHPLC) separations were performed on a Phenomenex Luna C18 10 μm, 250 × 30.0 mm column. Standard conditions were used for elution of all compounds, unless otherwise indicated, at a flow rate of 40 ml min −1 : 100% A to 100% B linear gradient over 15 min, followed by a further 10 min at 100% B where solvent B was 90% MeCN, 10% H 2 O±0.1% TFA and solvent A was H 2 O±0.1% TFA. Compounds were detected by ultraviolet absorption and pure fractions were lyophilized. Analytical rpHPLC was used to assess compound purity (Phenomenex Luna C18 column, 5 μm, 90 Å, 4.6 × 250 mm, at three different wavelengths λ =214, 230 and 254 nm). Standard conditions (same as preparative-scale rpHPLC) were used for all compounds, unless otherwise indicated, at a flow rate of 1 ml min −1 . Solvents were the same as for preparative-scale rpHPLC. All final compounds were ≥95% pure by analytical HPLC. Electrospray ionization mass spectra measurements were obtained on Micromass LCT. HRMS measurements were obtained on a Bruker microTOF mass spectrometer equipped with a Dionex LC system (Chromeleon) in positive ion mode by direct infusion in MeCN at 100 μl h −1 using sodium formate clusters as an internal calibrant. Data were processed using Bruker Daltonics DataAnalysis 3.4 software. Mass accuracy was consistently better than 1 p.p.m. error. 1 H and 13 C NMR spectra were recorded on Bruker Avance 600 or Varian 400 spectrometers at 298 K in the deuterated solvents indicated and were referenced to the residual 1 H signals; DMSO-d 6 2.50 p.p.m. and CD 3 OD 3.31 p.p.m., except CDCl 3 solutions were referenced to internal tetramethylsilane (TMS). The exact concentration of the compounds was determined by the quantitative NMR integration ‘PULCON’ experiment [45] . These settings were used for all PULCON experiments: relaxation delay of 30 s, 64 scans, 2 dummy scans, 90° pulse and temperature at 298 K. Synthesis of 3-indole-(Leu–Imidazole)–arg ( 16 ) Cbz–Leu–5-methylimidazole ethyl ester (0.24 g, 0.6 mmol) in MeOH (20 ml) was treated with 10% Pd/C (20 mg) and hydrogenated at 40 psi on a Parr hydrogenator for 5 h. The mixture was filtered through celite and the filtrate was concentrated in vacuo . The crude product was added to N -Boc-indole-3-carboxylic acid (0.20 g, 0.70 mmol), pre-activated (with O-(Benzotriazol-1-yl)-N,N,N′,N′-tetramethyluronium hexafluorophosphate, diisopropylethylamine in dimethylformamide 2 ml) and stirred overnight at room temperature. The reaction mixture was diluted with ethyl acetate and washed with saturated NaHCO 3 . The organic extracts were dried over MgSO 4 , filtered and concentrated in vacuo. The crude product was dissolved in ethyl alcohol/H 2 O/2 M NaOH (4:1:1, 3 ml) and heated in a microwave at 120 °C for 10 min. The ethyl alcohol in the reaction was removed in vacuo and the aqueous solution was acidified with 2 M HCl and extracted with ethyl acetate. The combined organic extracts were dried over MgSO 4 , filtered and concentrated in vacuo . The crude product was coupled to H–Arg–OEt and then the ester was hydrolysed with NaOH. The product was purified by rpHPLC and lyophilized to afford a white powder (20 mg, 7%). 1 H NMR (600 MHz, DMSO-d 6 ), δ 8.25 (br s, 1H), 8.17 (t, J =3.0 Hz, 1H), 8.12 (d, J =7.7 Hz, 1H), 8.02 (br s, 1H), 7.59 (br s, 1H), 7.44 (d, J =7.7 Hz, 1H), 7.15 (t, J =7.8 Hz, 1H), 7.10 (t, J =7.6 Hz, 1H), 5.36 (m, 1H), 4.41 (m, 1H), 3.17–3.08 (m, 2H), 2.43 (s, 3H), 1.96–1.82 (m, 2H), 1.80–1.63 (m, 3H), 1.56–1.49 (m, 2H), 0.96–0.92 (two sets of d, J =6.6 Hz, 6H). 13 C NMR (150 MHz, DMSO-d 6 ): δ 173.3, 164.5, 158.7, 158.5, 158.3, 156.6, 136.3, 128.7, 126.3, 122.0, 120.9, 120.5, 111.9, 51.2, 44.5, 42.0, 40.3, 28.5, 25.3, 24.4, 22.8, 21.6, 10.5. HRMS ( m/z ): [MH] + calcd for C 25 H 35 N 8 O 4 + , 511.2776; found, 511.2774; t R =7.9 min (0–100% B in 10 min gradient). Synthesis of 3-indole–(Leu–Ox)–arg ( 17 ) This compound was synthesized following the same procedure for compound 16 , except that H–Leu–Ox–OMe (0.11 g, 0.46 mmol) was used for coupling to N -Boc-indole-3-carboxylic acid and gave 17 ( 27 mg, 12%). 1 H NMR (600 MHz, DMSO-d 6 ): δ 8.59 (s, 1H), 8.39 (d, J =8.6 Hz, 1H), 8.22 (d, J =8.6 Hz, 1H), 8.16 (d, J =3.0 Hz, 1H), 8.11 (d, J =7.9 Hz, 1H), 7.55 (t, J =5.8 Hz, 1H), 7.43 (d, J =8.2 Hz, 1H), 7.15 (t, J =7.4 Hz, 1H), 7.09 (t, J =7.6 Hz, 1H), 5.36 (m, 1H), 4.40 (m, 1H), 3.14–3.06 (m, 2H), 1.96 (m, 1H), 1.87 (m, 1H), 1.83–1.75 (m, 2H), 1.69 (m, 1H), 1.56–1.45 (m, 2H), 1.00–0.91 (two sets of d, J =6.6 Hz, 6H); 13 C NMR (150 MHz, DMSO-d 6 ): δ 173.5, 165.5, 164.8, 160.5, 157.1, 142.5, 136.5, 135.8, 128.8, 126.7, 122.4, 121.4, 120.9, 112.3, 110.0, 51.6, 45.2, 41.7, 40.8, 28.3, 25.8, 24.7, 23.3, 21.9. HRMS ( m/z ): [MH] + calcd for C 24 H 32 N 7 O 5 + , 498.2459; found, 498.2461.; t R =7.3 min (20–100% B in 10 min gradient). Calculations of H-bond interaction energy The geometry of the water–heterocycle H-bonded complex was optimized at the MP2/6-311++G(3d,3p) level using Gaussian 09. The H-bond interaction energy was the difference in energy of the complex from the sum of energies of water and heterocycle, calculated in isolation by the same method [43] . Intracellular calcium release assay HMDMs (5 × 10 4 cells per well) were added to a 96-well cleared-bottom black-wall assay plate (Corning) and incubated overnight at 37 °C. Before assay, the medium was removed and cells were incubated with dye-loading buffer (12 ml Hank’s balance salt solution (HBSS) buffer, 4 μM Fluo-3 AM, 25 μl Pluronic acid F-127 and 1% fetal bovine serum) for 1 h at 37 °C. Cells were then washed once with assay buffer (HBSS supplemented with 2.5 mM probenecid and 20 mM HEPES, pH 7.4). Compounds were dissolved in dimethyl sulphoxide (DMSO) to make a 10-mM stock solution, then further diluted with HBSS buffer to the desired concentrations for intracellular calcium release assay. Fluorescence imaging plate reader was used to monitor intracellular release of Ca 2+ via fluorescence measurement (excitation 495 nm, emission 520 nm) for 5 min after injection of agonists. Changes in fluorescence (% response) were plotted against logarithmic concentrations of test compound. The EC 50 values were derived from concentration response curves using nonlinear regression in Graphpad Prism v5. 125 I-C3a radioligand binding assay Receptor binding was performed by ligand competition with 80 pM [ 125 I]-C3a (2,200 Ci mmol −1 ; Perkin Elmer, Torrance, CA, USA), HMDMs (1.2 × 10 6 cells ml −1 ), 80 pM [ 125 I]-C3a±various concentrations of unlabelled C3a or test agonist mixed with solvent (50 mM Tris, 3 mM MgCl 2 , 0.1 mM CaCl 2 , 0.5% (w/v) BSA, pH 7.4) for 60 min in a 96-well Nunc round-bottom plate at room temperature. Unbound [ 125 I]-C3a was removed by filtration through glass microfibre filter GF/B (Whatman Iner. Ltd, England), which had been soaked in 0.6% polyethyleneimine to reduce nonspecific binding. The filter was washed three times with cold buffer (50 mM Tris-HCl), pH 7.4, and bound [ 125 I]-C3a was assessed by scintillation counting on Microbeta counter. Specific [ 125 I]-C3a binding was defined as the difference between total binding and nonspecific binding as determined in the presence of 1 μM unlabelled C3a. The IC 50 value was derived from the concentration of agonist/antagonist required to inhibit 50% of [ 125 I]-C3a binding. Gene analysis HMDMs were seeded at 1 × 10 6 per ml and allowed to adhere overnight. For inhibition experiments, HMDMs were pretreated with Gαi inhibitor (200 ng ml −1 pertussis toxin, overnight) or PLCβ inhibitor (10 μM U73122, 30 min), or C3aR antagonist (10 μM SB290157, 30 min), before adding C3a or 17 (0.3 μM, 30 min). RNA was extracted from HMDMs according to ISOLATE II RNA Mini Kit (Bioline). Real-time PCR was measured on a ABI PRISM 7900HT instrument (Applied Biosystems), each target gene was normalized to housekeeping 18S rRNA and fold change was calculated relative to untreated control. Primer sequence is shown in Supplementary Table S1 . Isolation of HMDMs HMDMs were isolated using Ficoll-paque density centrifugation (GE Healthcare Bio-Science, Uppsala, Sweden) from buffy coat of anonymous human donors provided by the Australian Red Cross Blood Service, Brisbane. CD14 + monocytes were positively selected using CD14 + MACS magnetic beads (Miltenyi Biotech, Auburn, CA, USA) after successive magnetic sorting and washings. The CD14 + monocytes were then cultured at 37 °C with 5% CO 2 and differentiated to HMDMs using 100 ng ml −1 of recombinant human macrophage colony-stimulating factor (PeptroTech Inc., Rocky Hill, NJ, USA) at 1.5 × 106 cells per ml. HMDMs were kept in Iscove’s modified Dulbecco’s media supplemented with 10% fetal bovine serum, penicillin (10 U ml −1 ), streptomycin (10 U ml −1 ) and L -glutamine (2 mM; Invitrogen). HMDMs were supplemented after 5 days with fresh medium containing 100 ng ml −1 macrophage colony-stimulating factor. HMDMs were collected by gentle scraping in saline solution on day 7. β-Hexosaminidase release assay LAD2 human mast cells (kindly provided by Dr Dean Metcalfe, National Institute of Allergy and Infectious Diseases, National Institute of Health) were cultured as previously described [46] and β-hexosaminidase release assay was performed as reported [47] . Briefly, LAD2 cells were presensitized with IgE (100 ng ml −1 ) overnight before experiment. In the antagonist assay, SB290157 was pre-incubated for 30 min before the addition of C3a or 17, and release of β-hexosaminidase was measured at 405 nm using FLUOstar Optima (BMG LabTechnologies). How to cite this article: Reid, R. C. et al. Downsizing a human inflammatory protein to a small molecule with equal potency and functionality. Nat. Commun. 4:2802 doi: 10.1038/ncomms3802 (2013).